Hepatic IRE1α regulates fasting-induced metabolic adaptive programs through the XBP1s–PPARα axis signalling Although the mammalian IRE1α-XBP1 branch of the cellular unfolded protein response has been implicated in glucose and lipid metabolism, the exact metabolic role of IRE1α signalling in vivo remains poorly understood. Here we show that hepatic IRE1α functions as a nutrient sensor that regulates the metabolic adaptation to fasting. We find that prolonged deprivation of food or consumption of a ketogenic diet activates the IRE1α-XBP1 pathway in mouse livers. Hepatocyte-specific abrogation of Ire1 α results in impairment of fatty acid β-oxidation and ketogenesis in the liver under chronic fasting or ketogenic conditions, leading to hepatosteatosis; liver-specific restoration of XBP1s reverses the defects in IRE1α null mice. XBP1s directly binds to and activates the promoter of PPARα, the master regulator of starvation responses. Hence, our results demonstrate that hepatic IRE1α promotes the adaptive shift of fuel utilization during starvation by stimulating mitochondrial β-oxidation and ketogenesis through the XBP1s–PPARα axis. In eukaryotes, accumulation of unfolded or misfolded proteins in the endoplasmic reticulum (ER) lumen causes ER stress, activating the cellular unfolded protein response (UPR) [1] , [2] . Three canonical branches of the UPR are governed by the ER-resident signal transducers, inositol-requiring enzyme 1 (IRE1), PKR-like endoplasmic reticulum kinase (PERK) and activating transcription factor 6 (ATF6) [1] , [2] . IRE1 is the most conserved ER stress sensor that possesses both Ser/Thr kinase and RNase activities [2] . On activation through trans-autophosphorylation and dimerization/oligomerization [2] , [3] , [4] , IRE1 catalyses the non-conventional splicing of the mRNA-encoding X-box-binding protein 1 (XBP1), thereby producing an active spliced form of this transcription factor (XBP1s) to initiate a key UPR programme [5] . In mammals, changes of metabolic cues are also able to activate the IRE1α and other UPR pathways [6] , [7] , [8] , [9] , [10] . Perturbation of ER homoeostasis is thought to represent an important mechanism underlying metabolic dysregulation [11] , [12] . Studies in animal models have implicated IRE1α or XBP1s in both glucose and lipid metabolism [6] , [8] , [9] , [13] , [14] , [15] , [16] , [17] , [18] , [19] , [20] . Recently, it was shown that the hepatic IRE1α-XBP1 pathway is activated upon refeeding, and overexpression of XBP1s in livers of mice may promote postprandial metabolic changes [6] . Hepatic overexpression of XBP1s was also reported to exert a suppressive effect upon gluconeogenesis [15] , [20] . In addition, the hepatic IRE1α-XBP1 pathway was shown to play a crucial role in the assembly of very low-density lipoprotein (VLDL) and hepatic lipid homoeostasis through regulation of protein disulphide isomerase expression [18] . Despite these recent progresses, it remains largely elusive how IRE1α acts under physiological conditions through the Xbp1 mRNA-splicing event to regulate metabolic pathways. Previously we demonstrated that glucagon can stimulate the phosphorylation by PKA of IRE1α in mouse hepatocytes, which promotes the gluconeogenic programme upon acute fasting [8] . Given that the liver performs multiple metabolic functions during the periods of fasting and starvation, we investigated the activation and function in vivo of the hepatic IRE1α-XBP1 pathway during the adaptive shift of fuel utilization in response to nutrient deprivation. We found that the hepatic IRE1α-XBP1 pathway is activated in mice during prolonged fasting or by a ketogenic diet (KD), and hepatocyte-specific deletion of IRE1α impairs fatty acid β-oxidation and ketogenesis. Futhermore, IRE1α regulates this metabolic adaptation process through XBP1s-mediated upregulation of PPARα expression. Our findings reveal a key role for hepatic IRE1α as a metabolic sensor in the starvation responses. Chronic fasting activates the hepatic IRE1α-XBP1 pathway We first examined the activation of the IRE1α-XBP1 pathway in the liver of mice that were subjected to a short (6 h) or a long period (18 h) of fasting. Both conditions of fasting similarly stimulated Ser 724 phosphorylation of IRE1α in the liver ( Fig. 1a ). Phos-tag gel [21] , [22] analyses showed a slightly higher mobility shift of IRE1α protein upon prolonged fasting than that under short-term fasting, suggesting a higher extent of phosphorylation of hepatic IRE1α during the extended period of food deprivation ( Fig. 1b ). Prolonged fasting also increased Xbp1 mRNA splicing (by approximately 4-fold) ( Fig. 1c ) and nuclear accumulation of XBP1s protein in the livers ( Fig. 1d ); by contrast, short-term fasting was unable to increase Xbp1 mRNA splicing. Chronic fasting did not activate the PERK-eIF2α or ATF6α branch of the UPR ( Fig. 1a ), indicating that nutrient deprivation specifically stimulated the IRE1α-XBP1 pathway. Next, we generated liver-specific IRE1α knockout (referred to as LKO) mice using the Cre/ loxP system ( Supplementary Fig. 1 ). We observed that hepatocyte-specific deletion of IRE1α completely abolished fasting-induced increases in nuclear XBP1s proteins in LKO mice ( Fig. 1e ). Fasting also increased the expression of ERdj4 and Sec61 α, two XBP1-target genes, in flox/flox but not LKO mice ( Supplementary Fig. 2a ). Notably, abrogation of the hepatic IRE1α-XBP1 pathway did not affect liver expression of FAS and ACC1, two key lipogenic enzymes, in either fed or fasted LKO mice ( Fig. 1e ; Supplementary Fig. 2b ). To further verify activation of the hepatic IRE1α-XBP1 pathway by chronic fasting, we introduced an Xbp1 -splicing-directed luciferase reporter [23] into the livers of mice through hydrodynamic injection [24] . Consistently, in comparison with a 6-h short-term fast or ad libitum feeding, prolonged fasting for 18 h induced a marked elevation of liver luciferase reporter activity in flox/flox mice, but not in LKO mice ( Fig. 1f ). These results demonstrate a catabolic mode of activation of the Xbp1 -splicing activity of IRE1α in response to extended periods of food deprivation. 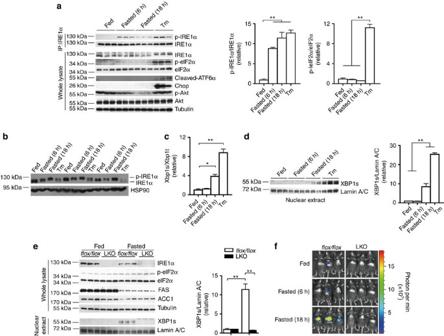Figure 1: Prolonged food deprivation results in activation of the IRE1α-XBP1 pathway in the liver. (a–d) Male C57BL/6 mice were fedad libitumor denied food for 6 or 18 h (n=5 per group) before being killed at the same time of the day. Mice i.p. injected with tunicamycin (Tm, 2 mg kg−1body weight) was used as a control group. (a) Immunoblotting of liver extracts immunoprecipitated with the IRE1α antibody or total liver lysates using the indicated antibodies, and representative results are shown for three individual mice per group. Relative phosphorylation levels of IRE1α and eIF2α were determined by densitometric quantification of the immunoblots, presented as the mean±s.e.m. (n=3). **P<0.01 by one-way analysis of variance (ANOVA). (b) Phos-tag gel analysis of IRE1α phosphorylation from total liver lysates. HSP90 was used as a loading control. (c) Analysis of liverXbp1mRNA splicing by quantitative real-time RT–PCR. Results were normalized to the value of the fed group and are shown as the mean±s.e.m. (n=5). *P<0.05, **P<0.01 by one-way ANOVA. (d) Immunoblotting of liver nuclear extracts using the indicated antibodies. Relative XBP1s levels were determined by densitometric quantification of the immunoblots, shown as the mean±s.e.m. (n=3). *P<0.05, by one-way ANOVA. (e) Male liver-specific IRE1α knockout mice (LKO) and age-matchedflox/floxlittermates were fedad libitumor subjected to an 18-h fast. Total liver lysates and nuclear extracts were analysed by immunoblotting using the indicated antibodies. Relative nuclear XBP1s levels were quantified and presented as the mean±s.e.m. (n=3). **P<0.01 by two-way ANOVA. (f) Age-matched male LKO andflox/floxmice were engineered to express anXbp1-splicing-Luc reporter in livers. Luciferase activities were monitoredin vivoby the imaging system under the indicated fed or fasted states. Representative results are shown for three individual mice per group. Figure 1: Prolonged food deprivation results in activation of the IRE1α-XBP1 pathway in the liver. ( a – d ) Male C57BL/6 mice were fed ad libitum or denied food for 6 or 18 h ( n =5 per group) before being killed at the same time of the day. Mice i.p. injected with tunicamycin (Tm, 2 mg kg −1 body weight) was used as a control group. ( a ) Immunoblotting of liver extracts immunoprecipitated with the IRE1α antibody or total liver lysates using the indicated antibodies, and representative results are shown for three individual mice per group. Relative phosphorylation levels of IRE1α and eIF2α were determined by densitometric quantification of the immunoblots, presented as the mean±s.e.m. ( n =3). ** P <0.01 by one-way analysis of variance (ANOVA). ( b ) Phos-tag gel analysis of IRE1α phosphorylation from total liver lysates. HSP90 was used as a loading control. ( c ) Analysis of liver Xbp1 mRNA splicing by quantitative real-time RT–PCR. Results were normalized to the value of the fed group and are shown as the mean±s.e.m. ( n =5). * P <0.05, ** P <0.01 by one-way ANOVA. ( d ) Immunoblotting of liver nuclear extracts using the indicated antibodies. Relative XBP1s levels were determined by densitometric quantification of the immunoblots, shown as the mean±s.e.m. ( n =3). * P <0.05, by one-way ANOVA. ( e ) Male liver-specific IRE1α knockout mice (LKO) and age-matched flox/flox littermates were fed ad libitum or subjected to an 18-h fast. Total liver lysates and nuclear extracts were analysed by immunoblotting using the indicated antibodies. Relative nuclear XBP1s levels were quantified and presented as the mean±s.e.m. ( n =3). ** P <0.01 by two-way ANOVA. ( f ) Age-matched male LKO and flox/flox mice were engineered to express an Xbp1 -splicing-Luc reporter in livers. Luciferase activities were monitored in vivo by the imaging system under the indicated fed or fasted states. Representative results are shown for three individual mice per group. Full size image IRE1α deficiency disrupts β-oxidation and ketogenesis The fasting-responsive activation of the hepatic IRE1α-XBP1 pathway prompted us to examine the metabolic role of IRE1α using the LKO mice, particularly in the state of prolonged fasting that evokes complex adaptive responses in fuel metabolism. During extended periods of food deprivation, the liver is known to undergo metabolic reprogramming to oxidize fatty acids and produce ketone bodies as the primary energy source for the brain. LKO mice exhibited normal body weight, food intake and glucose tolerance ( Supplementary Fig. 3a–d ), but they displayed massive accumulation of lipids ( Fig. 2a ) and markedly increased content of triglycerides (TGs) in the liver after prolonged fasting for 18 h ( Fig. 2b ). Interestingly, chronically fasted LKO mice had significant decreases in the serum levels of TG, free fatty acids (FFAs) and the ketone body β-hydroxybutyrate ( Fig. 2c–e ), indicating possible defects in TG secretion, adipocyte lipolysis and ketogenic output. As the de novo lipogenic programme was not altered in the livers of LKO animals ( Fig. 1e ; Supplementary Fig. 2b ), we asked if IRE1α deficiency could cause impairments in fatty acid oxidation, ketogenesis, and/or TG secretion. Indeed, relative to their flox/flox counterparts, liver extracts from fasted LKO mice had significantly reduced β-oxidation activity ( Fig. 2f ). Fasted LKO animals also showed a severe impairment in their ability to produce β-hydroxybutyrate ( Fig. 2g ) when given octanoate, a mitochondrion-permeable ketogenic substrate [25] , [26] . In addition, fasted LKO mice had lower serum levels of VLDL-TG ( Supplementary Fig. 3e ) and showed impaired hepatic VLDL secretion ( Supplementary Fig. 3f ), supporting the role of the IRE1α pathway in hepatic VLDL assembly and secretion that was recently reported [18] . Furthermore, we observed a pronounced reduction in the level of circulating fibroblast growth factor 21 (FGF21) in fasted LKO animals ( Fig. 2h ), a liver-secreted hormone that has critical roles in lipid homoeostasis during starvation [27] , [28] , [29] . Given that FGF21 is a key endocrine regulator of adipocyte lipolysis [28] , this may account for, at least partially, the decreased levels of circulating FFAs in fasted LKO mice ( Fig. 2d ). We then tested if IRE1α ablation affected the expression of peroxisome proliferator-activated receptor α (PPARα), the master nuclear receptor regulator that orchestrates the gene expression programs in response to starvation [30] , [31] , [32] . Liver gene expression profiling revealed that disruption of fasting-stimulated Xbp1 mRNA splicing in LKO mice correlated with significant blunting of fasting-induced upregulation of Ppar α but not Ppar γ ( Fig. 2i ). Conversely, overexpression of the wild-type IRE1α, but not the K599A or K907A mutant [9] , increased Xbp1 mRNA splicing and the expression of Ppar α in primary LKO hepatocytes ( Fig. 3a–c ). Consistently, we detected a significant reduction in fasting-induced expression of PPARα-target genes in LKO livers, including Fgf21 as well as peroxisomal acyl-CoA oxidase1 ( Acox1 ), carnitine palmitoyltransferase 1a ( Cpt1a ) and hydroxymethylglutaryl-CoA synthase ( Hmgcs2 ) ( Fig. 2i ), critical enzymes in β-oxidation and ketogenesis. Together, these data suggest a crucial role for hepatic IRE1α in promoting prolonged fasting-induced fatty acid β-oxidation and ketogenesis through influencing PPARα-dependent gene expression programs, in addition to regulating VLDL assembly and secretion [18] . 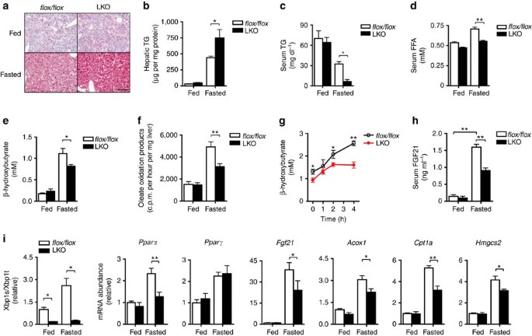Figure 2: Abrogation of hepatic IRE1α impairs fasting-induced fatty acid β-oxidation and ketogenesis. Male LKO mice and age-matchedflox/floxlittermates were fedad libitumor fasted for 18 h (n=6 per group). (a) Representative liver sections stained with Oil-red O (scale bar, 50 μm). (b) Liver content of TGs. (c–e) Serum levels of (c) TG, (d) FFAs and (e) β-hydroxybutyrate. (f) Fatty acid β-oxidation was determined using fresh liver homogenates. (g) Fasted mice were injected i.p. with sodium octanoate (0.5 mg per kg body weight). Serum β-hydroxybutyrate was measured from tail-vein blood at the indicated time points. (h) Serum levels of FGF21. (i) Analyses of hepaticXbp1mRNA splicing and the mRNA abundance of the indicated genes by quantitative RT–PCR using actin as the internal control. All data are shown as the mean±s.e.m. (n=6). *P<0.05, **P<0.01 by two-way analysis of variance inb–fandh–i, or byt-test ing. Figure 2: Abrogation of hepatic IRE1α impairs fasting-induced fatty acid β-oxidation and ketogenesis. Male LKO mice and age-matched flox/flox littermates were fed ad libitum or fasted for 18 h ( n =6 per group). ( a ) Representative liver sections stained with Oil-red O (scale bar, 50 μm). ( b ) Liver content of TGs. ( c – e ) Serum levels of ( c ) TG, ( d ) FFAs and ( e ) β-hydroxybutyrate. ( f ) Fatty acid β-oxidation was determined using fresh liver homogenates. ( g ) Fasted mice were injected i.p. with sodium octanoate (0.5 mg per kg body weight). Serum β-hydroxybutyrate was measured from tail-vein blood at the indicated time points. ( h ) Serum levels of FGF21. ( i ) Analyses of hepatic Xbp1 mRNA splicing and the mRNA abundance of the indicated genes by quantitative RT–PCR using actin as the internal control. All data are shown as the mean±s.e.m. ( n =6). * P <0.05, ** P <0.01 by two-way analysis of variance in b – f and h – i , or by t -test in g . 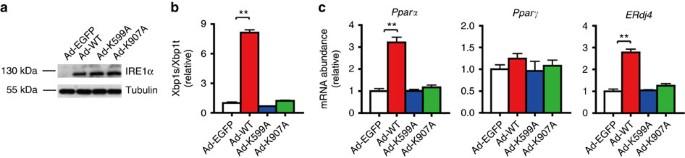Figure 3: Effects of overexpressed IRE1α proteins on the expression ofPparα. Primary hepatocytes from male LKO mice were infected for 2 days with adenoviruses expressing EGFP or the indicated human IRE1α proteins. (a) Immunoblotting analysis of the IRE1α protein expression. (b,c) Quantitative RT–PCR analyses of (b)Xbp1mRNA splicing and (c) the mRNA abundance of the indicated genes. Data are presented as the mean±s.e.m. (n=3 independent experiments). **P<0.01 by one-way analysis of variance. Full size image Figure 3: Effects of overexpressed IRE1α proteins on the expression of Ppar α. Primary hepatocytes from male LKO mice were infected for 2 days with adenoviruses expressing EGFP or the indicated human IRE1α proteins. ( a ) Immunoblotting analysis of the IRE1α protein expression. ( b , c ) Quantitative RT–PCR analyses of ( b ) Xbp1 mRNA splicing and ( c ) the mRNA abundance of the indicated genes. Data are presented as the mean±s.e.m. ( n =3 independent experiments). ** P <0.01 by one-way analysis of variance. Full size image IRE1α mediates the metabolic actions of glucagon and FFAs Prolonged fasting caused sustained increases in the levels of circulating glucagon and FFAs ( Fig. 4a ), which have been shown to stimulate the UPR responses [8] , [12] . We considered that FFAs and glucagon may mediate the fasting-induced activation of the hepatic IRE1α-XBP1 pathway. In agreement, glucagon or FFAs stimulated Xbp1 mRNA splicing in primary mouse hepatocytes; interestingly, glucagon and FFAs together stimulated Xbp1 mRNA splicing in a synergistic fashion ( Fig. 4b ), leading to increased nuclear accumulation of XBP1s protein ( Fig. 4c ). Notably, glucagon plus FFAs stimulated the phosphoryation of IRE1α but did not induce the activation of the PERK-eIF2α or ATF6α pathway ( Fig. 4d ), similar to the observations in fasted mouse livers ( Fig. 1a ). Moreover, glucagon plus FFAs could enhance fatty acid β-oxidation and ketogenesis in hepatocytes ( Fig. 4e,f ). Hepatocyte-specific deletion of IRE1α significantly deceased the ability of glucagon plus FFAs to stimulate β-oxidation ( Fig. 4e ), ketogenesis ( Fig. 4f ) and expression of Ppar α and Fgf21 ( Fig. 4g ). These results suggest that hepatic IRE1α promotes the β-oxidation and ketogenesis programs during starvation by integrating both nutrient (e.g., FFAs) and hormonal signals (e.g., glucagon). 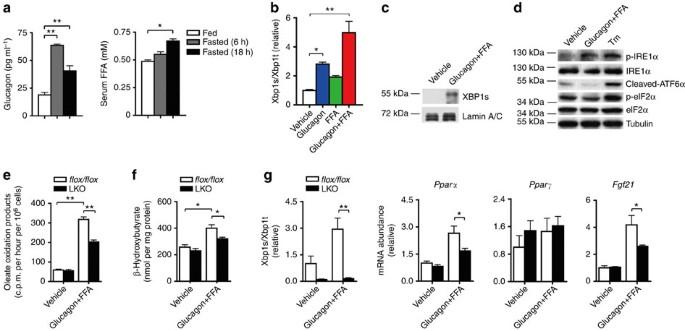Figure 4: Hepatic IRE1α deficiency blunts the stimulation of β-oxidation and ketogenesis by glucagon and FFAs. (a) Serum concentrations of glucagon and FFAs were measured in fed or fasted mice as indicated. Results are shown as the mean±s.e.m. (n=5). *P<0.05, **P<0.01 by one-way analysis of variance. (b) Primary hepatocytes isolated from male C57BL/6 mice were treated with 100 nM glucagon for 12 h, or 0.4 mM FFA mixture (0.1 mM palmitate, 0.1 mM oleate, 0.1 mM stearate and 0.1 mM linoleate) in 0.4% BSA (that is, FFA/BSA at a molar ratio of 6) for 6 h, or a combination of treatment with glucagon for 12 h and FFA mixture for 6 h. PBS or 0.4% BSA was used as the respective vehicle control for glucagon or the FFA mixture.Xbp1mRNA splicing was analysed by quantitative RT–PCR. Results are presented as the mean±s.e.m. (n=3 independent experiments). *P<0.05, **P<0.01 by one-way analysis of variance. (c) Immunoblotting of nuclear XBP1s protein in hepatocytes treated with glucagon plus FFAs. (d) Primary hepatocytes were treated with glucagon plus FFA mixture or with tunicamycin (5 μg ml−1) for 2 h. Cell lysates were analysed by immunoblotting using the indicated antibodies. Data are representative of three independent experiments. (e–g) Hepatocytes from male LKO andflox/floxmice were treated with glucagon plus FFA mixture. (e) Fatty acid β-oxidation rates and (f) β-hydroxybutyrate production were measured. (g) Analyses ofXbp1mRNA splicing and the mRNA abundance ofPparα,Pparγ andFgf21by quantitative RT–PCR. Results are presented as the mean±s.e.m. (n=3 independent experiments). *P<0.05, **P<0.01 by two-way analysis of variance. Figure 4: Hepatic IRE1α deficiency blunts the stimulation of β-oxidation and ketogenesis by glucagon and FFAs. ( a ) Serum concentrations of glucagon and FFAs were measured in fed or fasted mice as indicated. Results are shown as the mean±s.e.m. ( n =5). * P <0.05, ** P <0.01 by one-way analysis of variance. ( b ) Primary hepatocytes isolated from male C57BL/6 mice were treated with 100 nM glucagon for 12 h, or 0.4 mM FFA mixture (0.1 mM palmitate, 0.1 mM oleate, 0.1 mM stearate and 0.1 mM linoleate) in 0.4% BSA (that is, FFA/BSA at a molar ratio of 6) for 6 h, or a combination of treatment with glucagon for 12 h and FFA mixture for 6 h. PBS or 0.4% BSA was used as the respective vehicle control for glucagon or the FFA mixture. Xbp1 mRNA splicing was analysed by quantitative RT–PCR. Results are presented as the mean±s.e.m. ( n =3 independent experiments). * P <0.05, ** P <0.01 by one-way analysis of variance. ( c ) Immunoblotting of nuclear XBP1s protein in hepatocytes treated with glucagon plus FFAs. ( d ) Primary hepatocytes were treated with glucagon plus FFA mixture or with tunicamycin (5 μg ml −1 ) for 2 h. Cell lysates were analysed by immunoblotting using the indicated antibodies. Data are representative of three independent experiments. ( e – g ) Hepatocytes from male LKO and flox/flox mice were treated with glucagon plus FFA mixture. ( e ) Fatty acid β-oxidation rates and ( f ) β-hydroxybutyrate production were measured. ( g ) Analyses of Xbp1 mRNA splicing and the mRNA abundance of Ppar α, Ppar γ and Fgf21 by quantitative RT–PCR. Results are presented as the mean±s.e.m. ( n =3 independent experiments). * P <0.05, ** P <0.01 by two-way analysis of variance. Full size image IRE1α deficiency results in defective ketone production We next examined the hepatic IRE1α pathway in two additional ketotic models: mice fed a high-fat, low-carbohydrate KD [27] , or treated with streptozotocin (STZ) to induce type 1 diabetes [33] . In comparison with feeding a normal chow diet, consumption of KD for 3 days markedly increased IRE1α phosphorylation and nuclear accumulation of XBP1s protein ( Fig. 5a ). KD feeding also augmented the Xbp1 -splicing Luc activity in the livers of flox/flox but not LKO mice ( Fig. 5b ). KD-fed LKO mice had higher levels of liver lipids ( Fig. 5c,d ) and lower levels of serum TG ( Fig. 5e ) and β-hydroxybutyrate ( Fig. 5f ) than flox/flox control mice. In parallel with abrogation of KD-stimulated Xbp1 mRNA splicing, KD-induced upregulation of Ppar α, as well as its target genes Fgf21, Cpt1a and Hmgcs2 , was significantly blunted in the livers of LKO mice ( Fig. 5g ). We also examined the ketone production associated with STZ-induced type 1 diabetes in flox/flox and LKO mice. STZ-treated mice developed hyperglycaemia, hypoinsulinemia and hyperglucagonemia along with increased serum TG and FFA levels ( Fig. 6a–e ). STZ treatment increased the serum level of β-hydroxybutyrate by >5-fold in flox/flox mice, and ablation of hepatic IRE1α decreased it by ~45% in STZ-treated LKO mice ( Fig. 6f ). Remarkably, STZ treatment resulted in an ~12-fold increase in hepatic Xbp1 mRNA splicing, along with significant upregulation of Ppar α and its target genes, in flox/flox mice but not in LKO mice ( Fig. 6g ). Together, these data indicate that the hepatic IRE1α pathway serves as a common route to promote ketogenesis by multiple physiological and pathological factors. 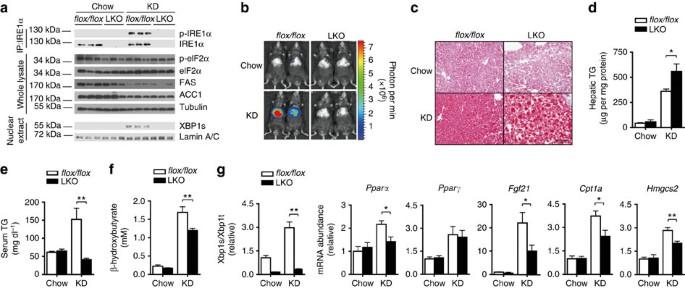Figure 5: Hepatic IRE1α ablation reduces diet-induced ketogenesis. Age-matched male mice of the indicated genotype were fed a normal chow or KD for 3 days. (a) Immunoblotting of liver extracts immunoprecipitated with the IRE1α antibody, total liver lysates and nuclear extracts. Representative results are shown for three individual mice. (b) Age-matched male mice were engineered to express theXbp1-splicing-Luc reporter in livers. Luciferase activities were monitoredin vivo. (c) Representative liver sections stained with Oil-red O (scale bar, 50 μm). (d) Liver TG content. (e,f) Serum levels of (e) TG and (f) β-hydroxybutyrate. (g) Quantitative RT–PCR analyses of hepaticXbp1mRNA splicing and the mRNA abundance of the indicated genes. Data ind–gare shown as the mean±s.e.m. (n=6). *P<0.05, **P<0.01 by two-way analysis of variance. Figure 5: Hepatic IRE1α ablation reduces diet-induced ketogenesis. Age-matched male mice of the indicated genotype were fed a normal chow or KD for 3 days. ( a ) Immunoblotting of liver extracts immunoprecipitated with the IRE1α antibody, total liver lysates and nuclear extracts. Representative results are shown for three individual mice. ( b ) Age-matched male mice were engineered to express the Xbp1 -splicing-Luc reporter in livers. Luciferase activities were monitored in vivo . ( c ) Representative liver sections stained with Oil-red O (scale bar, 50 μm). ( d ) Liver TG content. ( e , f ) Serum levels of ( e ) TG and ( f ) β-hydroxybutyrate. ( g ) Quantitative RT–PCR analyses of hepatic Xbp1 mRNA splicing and the mRNA abundance of the indicated genes. Data in d – g are shown as the mean±s.e.m. ( n =6). * P <0.05, ** P <0.01 by two-way analysis of variance. 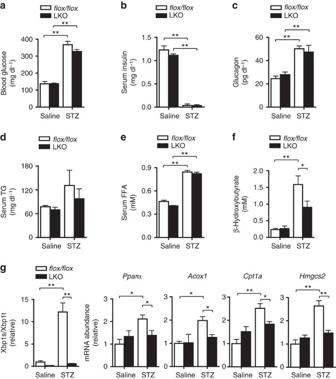Figure 6: Abrogation of hepatic IRE1α decreases ketone production in diabetic mice. Male LKO mice andflox/floxlittermates at 8–10 weeks of age were injected i.p. with saline or STZ (200 mg per kg body weight). (a) Blood glucose was measured at 3 days after treatment. (b–f) At 10 days after STZ treatment, mice were killed and serum levels of (b) insulin, (c) glucagon, (d) TG, (e) FFAs and (f) β-hydroxybutyrate were determined. (g) Quantitative RT–PCR analyses of hepaticXbp1mRNA splicing and mRNA abundance of the indicated genes. All data are shown as the mean±s.e.m. (n=6 per group). *P<0.05, **P<0.01 by two-way analysis of variance. Full size image Figure 6: Abrogation of hepatic IRE1α decreases ketone production in diabetic mice. Male LKO mice and flox/flox littermates at 8–10 weeks of age were injected i.p. with saline or STZ (200 mg per kg body weight). ( a ) Blood glucose was measured at 3 days after treatment. ( b – f ) At 10 days after STZ treatment, mice were killed and serum levels of ( b ) insulin, ( c ) glucagon, ( d ) TG, ( e ) FFAs and ( f ) β-hydroxybutyrate were determined. ( g ) Quantitative RT–PCR analyses of hepatic Xbp1 mRNA splicing and mRNA abundance of the indicated genes. All data are shown as the mean±s.e.m. ( n =6 per group). * P <0.05, ** P <0.01 by two-way analysis of variance. Full size image XBP1s normalizes the metabolic impairment in IRE1α null mice To determine whether XBP1s acts downstream of IRE1α to regulate β-oxidation and ketogenesis, we introduced recombinant XBP1s into the livers of LKO mice via adenoviral infection ( Fig. 7a ). Under chronic fasting, liver-specific expression of XBP1s decreased liver TG content ( Fig. 7b ) and increased serum β-hydroxybutyrate ( Fig. 7c ) in LKO mice to similar levels as in flox/flox control mice. Restoration of XBP1s also increased liver β-oxidation to normal levels in LKO mice ( Fig. 7d ). These metabolic changes were accompanied by reversal of the impairment in the fasting-induced expression of Ppar α ( Fig. 7e ) and its target genes, Fgf21 , Acox1 , Cpt1a and Hmgcs2 ( Fig. 7f ). Notably, exogenous XBP1s did not further enhance the expression of Ppar α and its target genes except Fgf21 in chronically fasted livers of flox/flox mice, which could be owing to the occurrence of fasting-induced nuclear accumulation of endogenous XBP1s ( Fig. 1e ). These results demonstrate that XBP1s directly mediates the metabolic effects of IRE1α upon β-oxidation and ketogenesis during chronic food deprivation. 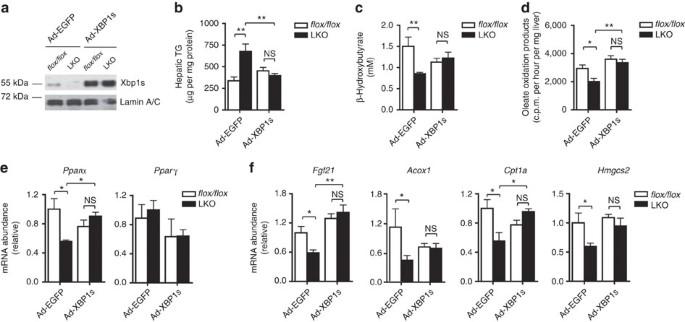Figure 7: Restored hepatic expression of XBP1s reverses the metabolic defects of LKO mice. Mice of the indicated genotype were infected with adenoviruses expressing EGFP or Flag-tagged XBP1s (n=6 per group) for 10 days and subsequently subjected to an 18-h fast. (a) Immunoblotting of liver nuclear extracts. (b) Liver TG content. (c) Serum level of β-hydroxybutyrate. (d) Fatty acid β-oxidation rates were determined using fresh liver homogenates. (e,f) Analyses by quantitative RT–PCR of hepatic mRNA abundance of (e)Pparα andPparγ and (f) the indicated PPARα-target genes. All data are shown as the mean±s.e.m. (n=6). *P<0.05, **P<0.01 by two-way analysis of variance. NS, no significance. Figure 7: Restored hepatic expression of XBP1s reverses the metabolic defects of LKO mice. Mice of the indicated genotype were infected with adenoviruses expressing EGFP or Flag-tagged XBP1s ( n =6 per group) for 10 days and subsequently subjected to an 18-h fast. ( a ) Immunoblotting of liver nuclear extracts. ( b ) Liver TG content. ( c ) Serum level of β-hydroxybutyrate. ( d ) Fatty acid β-oxidation rates were determined using fresh liver homogenates. ( e , f ) Analyses by quantitative RT–PCR of hepatic mRNA abundance of ( e ) Ppar α and Ppar γ and ( f ) the indicated PPARα-target genes. All data are shown as the mean±s.e.m. ( n =6). * P <0.05, ** P <0.01 by two-way analysis of variance. NS, no significance. Full size image Hepatic IRE1α controls the expression of Ppar α through XBP1s We then examined whether Ppar α is a direct transcriptional target of the IRE1α-XBP1 pathway. As overexpression of XBP1s in primary hepatocytes could increase the expression of Ppar α but not Ppar γ ( Fig. 8a ), we analysed the mouse Ppar α promoter and identified a putative UPR element (UPRE), a potential XBP1s-binding site [34] ( Fig. 8b ). Luciferase reporter assays showed that XBP1s directly stimulated the Ppar α promoter activity, and deletion of the putative UPRE abolished the ability of XBP1s to stimulate Ppar α promoter ( Fig. 8b ). To further determine whether XBP1s directly binds to the endogenous Ppar α promoter, we performed chromatin immunoprecipitation (ChIP) assays using nuclear extracts from primary hepatocytes overexpressing Flag-tagged XBP1s. Indeed, XBP1s physically bound to the putative UPRE-containing region of the Ppar α promoter ( Fig. 8c ). ChIP assays also revealed that this putative UPRE within the Ppar α promoter is required for XBP1s binding ( Fig. 8d ). Furthermore, fasting significantly increased the occupancy of the UPRE-containing region of the Ppar α promoter by endogenous XBP1s in the livers of flox/flox but not LKO mice ( Fig. 8e ). Consistently, imaging analyses of LKO mice with engineered Ppar α promoter-Luc reporter in their livers showed that hepatocyte-specific deletion of Ire1 α attenuated fasting-induced activation of the Ppar α promoter in animals ( Fig. 8f ). Thus, these results suggest that the IRE1α-XBP1 pathway promotes β-oxidation and ketogenesis by directly augmenting PPARα expression in the liver. 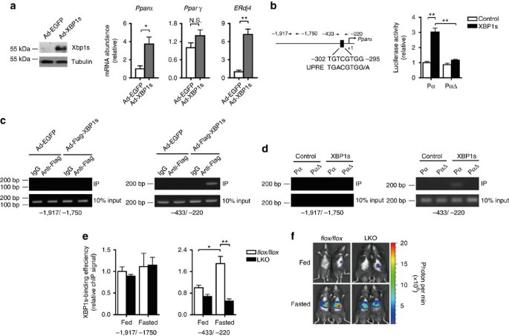Figure 8: Hepatic IRE1α promotes the expression ofPparα through XBP1s. (a) Primary hepatocytes from male C57BL/6 mice were infected for 2 days with adenoviruses expressing EGFP or Flag-tagged XBP1s protein. XBP1s protein was analysed by immunoblotting. Expression of the indicated genes was assessed by quantitative RT–PCR, and data are presented as the mean±s.e.m. (n=3 independent experiments). *P<0.05, **P<0.01 byt-test. (b) Schematic of thePparα promoter with the UPRE-like sequence indicated. Luciferase reporter assays were performed by co-transfection of 293T cells with the empty control vector or pCMV-XBP1s plasmid together with Luc constructs under the control of thePparα promoter (Pα) or that without the UPRE (PαΔ). Data are shown as the mean±s.e.m. (n=3 independent experiments). **P<0.01 by two-way analysis of variance. (c) Primary hepatocytes were infected with adenoviruses expressing EGFP or Flag-tagged XBP1s. Chromatin immunoprecipitaion (ChIP) was performed using control IgG or anti-Flag antibody prior to PCR amplification of the regions of thePparα promoter with (nucleotide −433 to −220) or without (nucleotide −1,917 to −1,750) the UPRE. (d) ChIP assays of extracts from 293T cells co-transfected with the empty control vector or pCMV-XBP1s plasmid together with the Pα or PαΔ reporter construct using anti-XBP1s antibody. (e) ChIP assays of liver nuclear extracts from male mice fedad libitumor fasted for 18 h using control IgG or anti-XBP1s antibody. Quantitative PCR results are shown as the mean±s.e.m. (n=6 per genotype). *P<0.05, **P<0.01 by two-way analysis of variance. (f) Age-matched male mice were engineered to express the Pα-Luc reporter in livers. Luciferase activities were monitoredin vivounder the indicated fed or fasted states. Figure 8: Hepatic IRE1α promotes the expression of Ppar α through XBP1s. ( a ) Primary hepatocytes from male C57BL/6 mice were infected for 2 days with adenoviruses expressing EGFP or Flag-tagged XBP1s protein. XBP1s protein was analysed by immunoblotting. Expression of the indicated genes was assessed by quantitative RT–PCR, and data are presented as the mean±s.e.m. ( n =3 independent experiments). * P <0.05, ** P <0.01 by t -test. ( b ) Schematic of the Ppar α promoter with the UPRE-like sequence indicated. Luciferase reporter assays were performed by co-transfection of 293T cells with the empty control vector or pCMV-XBP1s plasmid together with Luc constructs under the control of the Ppar α promoter (Pα) or that without the UPRE (PαΔ). Data are shown as the mean±s.e.m. ( n =3 independent experiments). ** P <0.01 by two-way analysis of variance. ( c ) Primary hepatocytes were infected with adenoviruses expressing EGFP or Flag-tagged XBP1s. Chromatin immunoprecipitaion (ChIP) was performed using control IgG or anti-Flag antibody prior to PCR amplification of the regions of the Ppar α promoter with (nucleotide −433 to −220) or without (nucleotide −1,917 to −1,750) the UPRE. ( d ) ChIP assays of extracts from 293T cells co-transfected with the empty control vector or pCMV-XBP1s plasmid together with the Pα or PαΔ reporter construct using anti-XBP1s antibody. ( e ) ChIP assays of liver nuclear extracts from male mice fed ad libitum or fasted for 18 h using control IgG or anti-XBP1s antibody. Quantitative PCR results are shown as the mean±s.e.m. ( n =6 per genotype). * P <0.05, ** P <0.01 by two-way analysis of variance. ( f ) Age-matched male mice were engineered to express the Pα-Luc reporter in livers. Luciferase activities were monitored in vivo under the indicated fed or fasted states. Full size image PPARα corrects the metabolic defects of IRE1α null mice To test if PPARα is the main metabolic effector of the hepatic IRE1α-XBP1 pathway, we overexpressed PPARα in the livers of LKO mice by adenoviral infection ( Fig. 9a ). Under prolonged fasting, forced expression of PPARα completely normalized the defective expression of its target genes Fgf21 , Acox1 , Cpt1a and Hmgcs2 in LKO livers ( Fig. 9b ). Moreover, PPARα overexpression in LKO mice significantly blunted their degrees of hepatic steatosis (from 66% increase of liver TG content in Ad-EGFP-infected control to 30% in Ad-PPARα-infected animals; Fig. 9c ), fully restored the serum levels of β-hydroxybutyrate ( Fig. 9d ), and completely corrected the impairment in liver β-oxidation ( Fig. 9e ). These data further demonstrate that hepatic IRE1α regulates fatty acid β-oxidation and ketogenesis through the XBP1s–PPARα axis. Notably, LKO mice with hepatic PPARα overexpression still showed significantly higher liver TG levels than Ad-EGFP-infected LKO mice ( Fig. 9c ). This indicates that metabolic defects arising from PPARα-independent mechanisms, for example, impairment of hepatic TG secretion ( Supplementary Fig. 3e,f ), also contributes to increased hepatic steatosis in LKO animals during chronic food deprivation. 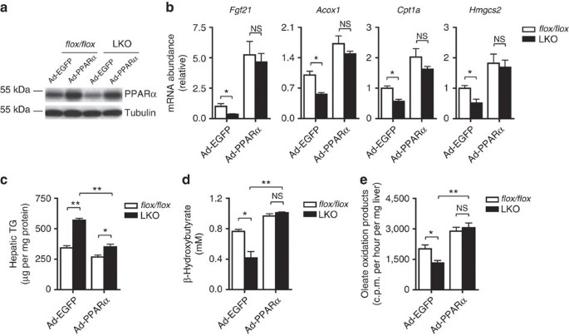Figure 9: Restored liver expression of PPARα normalized the metabolic defects of LKO mice. Mice of the indicated genotype were infected with adenoviruses expressing EGFP or PPARα for 5 days and subsequently subjected to an 18-h fast (n=5 per group). (a) Immunoblotting of liver nuclear extracts using the PPARα antibody. (b) Analyses by quantitative RT–PCR of hepatic mRNA abundance of the indicated PPARα-target genes. (c) Liver TG content. (d) Serum level of β-hydroxybutyrate. (e) Fatty acid β-oxidation rates were determined using fresh liver homogenates. All data are shown as the mean±s.e.m. (n=5). *P<0.05, **P<0.01 by two-way analysis of variance. NS, no significance. Figure 9: Restored liver expression of PPARα normalized the metabolic defects of LKO mice. Mice of the indicated genotype were infected with adenoviruses expressing EGFP or PPARα for 5 days and subsequently subjected to an 18-h fast ( n =5 per group). ( a ) Immunoblotting of liver nuclear extracts using the PPARα antibody. ( b ) Analyses by quantitative RT–PCR of hepatic mRNA abundance of the indicated PPARα-target genes. ( c ) Liver TG content. ( d ) Serum level of β-hydroxybutyrate. ( e ) Fatty acid β-oxidation rates were determined using fresh liver homogenates. All data are shown as the mean±s.e.m. ( n =5). * P <0.05, ** P <0.01 by two-way analysis of variance. NS, no significance. Full size image ATF6α does not affect β-oxidation and ketogenesis Because the UPR is known to manage ER stress by enhancing the ER protein-folding capacity [1] , [2] , we considered the possibility that the IRE1α-XBP1 pathway might exert its metabolic effects by inducing molecular chaperones such as BiP to improve ER functions. To test this, we examined the effects of ATF6α, the basic Leu zipper (bZIP) transcription factor which can enhance the expression of ER chaperones and may form a heterodimer with XBP1s [35] , [36] , upon the expression of Ppar α and lipid metabolism in hepatocytes. Overexpression of the full-length ATF6α in transfected 293T cells produced the active cleaved form of ATF6α [35] ( Supplementary Fig. 4a ). Similar to XBP1s, cleaved-ATF6α induced the expression of Bip ( Supplementary Fig. 4b ). By contrast, luciferase reporter assays showed that ATF6α could not activate the Ppar α promoter as XBP1s did ( Supplementary Fig. 4c ). Overexpression of ATF6α through hyperdynamic injection of animals with the ATF6α plasmid also generated cleaved-ATF6α protein in hepatocytes ( Supplementary Fig. 4d ), resulting in upregulation of Bip but not Ppar α ( Supplementary Fig. 4e ). Furthermore, ATF6α overexpression showed no reversing effects upon the reduction of β-oxidation and ketogenesis in LKO hepatocytes when stimulated by glucagon plus FFAs ( Supplementary Fig. 4f,g ). These results imply that the hepatic IRE1α-XBP1 pathway regulates the adaptive fasting response through upregulating Ppar α in a manner that is independent of enhancing ER functions. Under ER stress conditions, the IRE1α-XBP1 branch of the UPR plays a pivotal role in maintaining ER homoeostasis [1] . XBP1s, the potent transcription factor resulting from activation of the RNase activity of IRE1α, controls a key gene expression programme that copes with ER stress. Emerging evidence indicates that XBP1s also exerts its metabolic effects through regulating effector genes such as protein disulphide isomerase [18] or UDP-galactose-4-epimerase [6] , or through non-transcriptional actions such as promoting degradation of the Forkhead box O1 transcription factor [20] . Nonetheless, it remains largely nebulous how IRE1α integrates metabolic signals under physiological settings to execute its functions through generating the endogenous XBP1s protein. As illustrated by our schematic model ( Fig. 10 ), the current study reveals that hepatic IRE1α responds to catabolic cues (e.g., changes in hormones and metabolites) during extended periods of nutrient deprivation and modulates the mitochondrial β-oxidation and ketogenesis programs through the XBP1s–PPARα axis during the adaptive shift of fuel utilization. Our results demonstrate that the IRE1α-XBP1 branch of the UPR serves as an unanticipated mechanism that underlies the transcriptional induction of Ppar α in response to food deprivation [30] , [31] . Notably, Wang et al . [18] , [19] did not document changes in the expression of Ppar α in their liver-specific Ire1 α knockout mice, most likely due to the short period of fasting in the reported studies. In addition, liver microarray analyses by So et al . [17] in their liver-specific Xbp1 knockout mice also did not reveal expression changes in Ppar α target genes, which may be ascribable to the non-fasting conditions or owing to XBP1-deficiency-induced hyperactivation of IRE1α for its mRNA decay actions in this model. 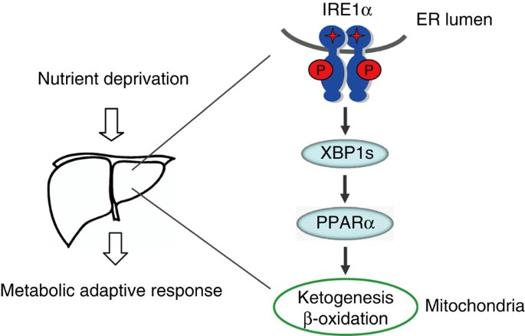Figure 10: Schematic model. During the adaptive shift of fuel utilization upon chronic nutrient deprivation, hepatic IRE1α serves as a catabolic sensor to regulate the β-oxidation and ketogenesis programs in mitochondria through the XBP1s–PPARα axis. Figure 10: Schematic model. During the adaptive shift of fuel utilization upon chronic nutrient deprivation, hepatic IRE1α serves as a catabolic sensor to regulate the β-oxidation and ketogenesis programs in mitochondria through the XBP1s–PPARα axis. Full size image It is intriguing that hepatic IRE1α can respond to both anabolic (e.g., refeeding) [6] and catabolic (e.g., food deprivation) states, in which distinct mechanisms may be involved in activating its Xbp1 mRNA-splicing activity. Upon refeeding, the increased workload of protein synthesis and folding within the ER presumably represents a metabolic state of ER stress; whereas upon chronic fasting, cytoplasmic signals emanating from catabolic cues (for example, glucagon and FFAs) may also drive the activation of the IRE1α-XBP1 pathway. Currently, it is unknown what different molecular features IRE1α may have during activation of its RNase activity for specific Xbp1 mRNA splicing under these two opposing metabolic states. It also has yet to be dissected how XBP1s can be delicately regulated in vivo to control different sets of gene expression programs under these circumstances. It warrants further investigation whether XBP1s may act as a molecular regulatory switch through acetylation [37] , phosphorylation [15] or other modifications under anabolic versus catabolic conditions. In summary, our findings indicate that hepatic IRE1α serves as a crucial component of the nutrient-sensing machinery that regulates the metabolic adaptive response to starvation. The identification of PPARα as a direct transcriptional target of XBP1s links the IRE1α-XBP1 branch of the UPR to the mitochondrial pathways in lipid metabolism. Given that excessive ER stress is associated with obesity-related metabolic dysregulation [8] , [12] , disruption of the IRE1α–XBP1s–PPARα cascade arising from perturbation of ER homoeostasis may provide an unappreciated mechanism that underlies mitochondrial dysfunction during the pathological progression of metabolic disorders. Animals C57BL/6J mice were purchased from Shanghai Laboratory Animal. Alb-Cre mice, which express the Cre recombinase transgene under the control of the Albumin promoter/enhancer elements, were generously provided by Dr Fudi Wang of the Institute for Nutritional Sciences, Chinese Academy of Sciences. To create liver-specific IRE1α knockout (LKO) mice, floxed mice in which the 121-nucleotide exon 2 of the Ern1 (that is, Ire1 α) allele was flanked with loxP recombination sites were generated at Shanghai Research Center for Model Organisms. After backcrossing into the genetic background of C57BL/6J, the Neo selection cassette was removed through crossing with FLP mice (129S4/SvJaeSor-Gt(ROSA)26Sortm1(FLP1)Dym/J, Jackson Lab). LKO mice ( Ire1 α f/f :Alb-Cre ) were subsequently produced by intercrossing Ire1 α f/f mice with the Alb-Cre mice. Animals were housed in laboratory cages at 23±3 °C with a humidity of 35±5% under a 12-h dark/light cycle (lights on at 6:30am), and were maintained on a regular chow diet (Shanghai Laboratory Animal Co. Ltd, Shanghai, China). Male mice between 8 and 14 weeks of age were used for all experiments. Mice fed ad libitum had free access to food and were killed after lights on for 2 h; fasted mice were denied food for 6 or 18 h and were killed at the same time of the day as the fed mice. For diet-induced ketogenesis studies, mice were fed ad libitum for 3 days a KD that contains 9.4% protein, 0.2% carbohydrate and 76.3% fat (w/w; Research Diets, Inc.), and were killed after lights on for 2 h. For diabetic ketoacidosis, mice were injected intraperitoneally (i.p.) with STZ (Sigma) at a dose of 200 mg kg −1 ; at 3 days after injection, mice with non-fasting blood glucose levels higher than 300 mg dl −1 were killed after lights on for 2 h for further analyses. All experimental protocols were approved by the Institutional Animal Care and Use Committee at the Institute for Nutritional Sciences, Shanghai Institutes for Biological Sciences, Chinese Academy of Sciences. Luciferase reporter analyses in vivo The luciferase (Luc) reporter plasmid for Xbp1 mRNA splicing was generously provided by Dr Masayuku Miura from RIKEN, Japan. The Luc reporter for the mouse Ppar α promoter spanning the region from −2,000 to +1 was constructed in pGL3 (Promega) utilizing a PCR-based cloning strategy. Reporter DNA constructs were introduced into livers of mice through hydrodynamic injection as described [24] . Briefly, a DNA solution (12.5 μg ml −1 in sterile PBS) was injected at 10% of volume/body weight through the tail vein within 10 s, and mice were then allowed to recover for 24 h. For in vivo imaging, anesthetized mice were injected i.p. with 1 mg per kg potassium luciferin (Promega), and images were captured after 5 min by the Live Animal Imaging System IVIS Lumina and analysed with Living Image software (Xenogen). Glucose and insulin tolerance tests After a fast of 6 h, mice were injected i.p. with 1 g per kg glucose or 0.75 U per kg insulin (Roche). Blood was collected by venous bleeding from the tail vein at 0, 15, 30, 60 and 90 min after the injection, and glucose concentrations were measured using a glucometer (FreeStyle). Oil-red O staining Frozen liver sections of 10 μm were fixed in formalin and then rinsed with 60% isopropanol. After staining with freshly prepared Oil-red O solution for 10 min, the sections were rinsed again with 60% isopropanol, and nuclei were stained with alum haematoxylin. Sections were analysed by inverted microscope (Olympus). Serum and liver measurements Serum levels of TGs, FFAs, β-hydroxybutyrate, insulin and glucagon were determined using the serum triglyceride determination kit (Sigma, triglyceride reagent T2449 and free glycerol reagent F6428), FFA assay kit (Cayman Chemical, 700310), β-hydroxybutyrate colorimetric assay kit (Cayman Chemical, 700190), insulin ELISA kit (Millipore, EZRMI-13K) and glucagon ELISA kit (BioVendor, RSCYK090R), respectively, all according to manufacturers’ instructions. Serum FGF21 was determined using ELISA kit (Millipore, EZRMFGF21-26K). For measurement of hepatic TGs, 40–50 mg of liver tissue was homogenized in 0.5 ml PBS. After sufficient mixing of 0.4-ml homogenates with 1.6 ml of CHCl 3 -CH 3 OH (2:1, v/v), the suspension was centrifuged at 3,000 r.p.m. for 10 min at room temperature. The lower organic phase was transferred and air-dried overnight in a chemical hood. The residual liquid was re-suspended in 800 μl of 1% Triton X-100 in absolute ethanol, and the concentration of TGs was determined using the serum triglyceride determination kit (Sigma, triglyceride reagent T2449 and free glycerol reagent F6428). Fatty acid β-oxidation assays To measure the activities of fatty acid β-oxidation from liver homogenates, 100 mg of fresh liver tissue was manually homogenized in 1 ml of ice-cold homogenization buffer (220 mM mannitol, 70 mM sucrose, 2 mM HEPES and 0.1 mM EDTA, pH 7.4), and 150 μl of homogenates were mixed with 850 μl of reaction buffer (50 mM EDTA, 150 mM Tris-HCl, 20 mM KH 2 PO 4 , 10 mM MgCl 2 -6H 2 O, 2 mM EDTA, 1 mM oleate complexed to fatty acid-free albumin at a molar ratio of 5:1, 0.3 μCi [9,10- 3 H(N)]-oleic acid, pH 7.4). After proceeding for 30 min at 37 °C, reactions were terminated by addition of 0.5 ml of 3 M perchloric acid. After incubation for 1 h at room temperature, precipitated protein was removed by centrifugation at the maximum speed, and 100 μl supernatant was mixed with 1 ml of scintillation liquid for radioactivity measurement using the liquid scintillation counter (Perkin Elmer). Reaction buffer that was treated likewise was used as the blank. To determine β-oxidation activities in hepatocytes, primary liver cells in 12-well plates were treated with FFA and glucagon as indicated, and washed with warm PBS. Cells were then incubated for 1 h at 37 °C in 0.25 ml of β-oxidation media (119 mM NaCl, 5 mM KCl, 2.6 mM KH 2 PO 4 , 2.6 mM MgSO 4 , 2 mM CaCl 2 , 24.6 mM NaHCO 3 , 10 mM HEPES, 8 mM oleate bound to fatty acid-free albumin at a molar ratio of 5:1 and 0.1 μCi [9,10- 3 H(N)]-oleic acid, pH 7.4), and 240 μl supernatant was subsequently transferred and mixed with 96 μl of 1.3 M perchloric acid. Precipitated protein was removed by centrifugation at the maximum speed, and 300 μl supernatant was mixed with 1 ml of scintillation liquid for radioactivity measurement. β-oxidation media treated likewise was used as the blank. Ketogenesis analyses To measure the ketogenic activities in vivo , mice were injected i.p. with 0.5 g kg −1 sodium octanoate (Sigma) after fasting for 18 h. Tail-vein blood was collected at 0, 1, 2 and 4 h after the injection, and serum β-hydroxybutyrate was measured using the β-hydroxybutyrate colorimetric assay kit (Cayman Chemical). To analyse ketogenesis in vitro , hepatocytes from mice of the desired genotype were incubated for 24 h in HepatoZYME-SFM (Gibco) medium containing 50 μM PPARα agonist WY-14643 (Cayman Chemical) and 2 mM sodium octanoate (Sigma). Aliquots of the media were then removed for measurement of β-hydroxybutyrate levels. Total cellular protein was determined and used for normalization. Measurement of hepatic TG secretion TG secretion rate from the liver was determined from mice after tail-vein injection of 600 mg kg −1 tyloxapol (Sigma) that inhibits the lipoprotein lipase activity. Serum TGs were measured from the tail vein blood at the desired time points. For lipoprotein analyses, equal volumes of serum were pooled for each group from individual mice (a total volume of 400 μl), and were fractionated using a Superose 6 10/300 GL FPLC column (Amersham Biosciences). Concentrations of TGs in each fraction (500 μl) were subsequently determined. Isolation of primary hepatocytes Hepatocytes were isolated from male mice at 8–12 weeks of age. Briefly, collagenase perfusion was performed through the portal vein of anesthetized mice with 50 ml of perfusion buffer (Krebs Ringer buffer containing 3.6 mg per ml glucose, 1 M CaCl 2 and 5,000 U of collagenase I (Worthington) at 37 °C. The liver was aseptically removed to a sterile 10-cm cell culture dish with 20 ml of ice-cold perfusion buffer without collagenase. The excised liver was cut and hepatocytes were dispersed by aspirating with a large-bore pipette, followed by filtration through a 70-μm cell strainer (Fisher) into a 50-ml centrifuge tube before centrifugation at 50g for 2 min at 4 °C. Cells were then washed with cold hepatocyte wash medium (Gibco) for three times and re-suspended in 15 ml of cold HepatoZYME-SFM (Gibco) medium supplemented with 2 mM L-glutamine, 20 units per ml penicillin and 20 μg per ml streptomycin. After the viability was determined by Trypan Blue staining, hepatocytes were plated at 6 × 10 5 cells per well in 6-well culture dishes or at 3 × 10 5 cells per well in 12-well dishes that were pre-coated with collagen. Cells were cultured for 8 h before further assays. Preparation of FFA mixture Palmitate, oleate, stearate or linoleate was each prepared as a 1 mM stock solution in 1% BSA in 1 mM NaOH at 60 °C. For treatment of hepatocytes with the FFA mixture, equal volumes of each fatty acid stock solution were mixed in HepatoZYME-SFM medium (Gibco) and used at the final concentration of 0.4 mM FFAs (0.1 mM for each of the four fatty acids) with 0.4% BSA (i.e., FFA/BSA at a molar ratio of 6) before use. BSA solution (0.4%) was used as the vehicle control. Adenovirus infection Recombinant adenoviruses for overexpression of EGFP and the wild-type or mutant forms of IRE1α were previously described [9] . The recombinant adenovirus for overexpression of the spliced form of XBP1 (XBP1s) was generously provided by Dr Ling Qi at Cornell University. For expression in hepatocytes, adenoviruses at an multiplicity of infection of 20–40 were used for infection. For liver XBP1s expression in mice, adenoviruses that were purified by two-step ultracentrifugation in cesium chloride gradient were used for tail-vein injection at ~5 × 10 8 plaque-forming units (p.f.u.) per mouse. Overexpression of ATF6α The pcDNA3.0-ATF6α plasmid was kindly provided by Dr Xu Shen from Shanghai Institute of Materia Medica, Chinese Academy of Sciences. For transient overexpression in HEK 293T cells, transfection was performed using Lipofectamine 2000 (Invitrogen) method according to the manufacturer’s instructions. For ATF6α expression in hepatocytes, plasmids were introduced into livers of mice by hydrodynamic injection through tail vein. Promoter reporter analyses The Ppar α promoter-luciferase reporter plasmid (Pα) and its deletion-mutant version (PαΔ) were constructed through a PCR-based strategy. For luciferase activity assays, 293T cells were co-transfected with the reporter plasmid, pCMV-XBP1s or pcDNA3.0-ATF6α plasmid and the β-galactosidase plasmid. Luciferase activity was determined using dual–luciferase reporter assay system (Promega) according to the manufacturer’s instructions, and β-galactosidase activity was used for normalization. Quantitative real-time RT–PCR Total RNA was isolated from liver tissues or hepatocytes using TRIzol reagent (Invitrogen), and cDNA was synthesized with M-MLV reverse transcriptase and random hexamer primers (Invitrogen). Real-time quantitative PCR was conducted with the SYBR Green PCR system (Applied Biosystems). β-Actin was utilized as an internal control for normalization. The oligonucleotide primers used are as follows: β-Actin : sense 5′-AGTGTGACGTTGACATCCGTA-3′, antisense 5′-GCCAGAGCAGTAATCTCCTTCT-3′; Xbp-1s : sense 5′-CTGAGTCCGAATCAGGTGCAG-3′, antisense 5′-GTCCATGGGAAGATGTTCTGG-3′; Xbp-1t : sense 5′-TGGCCGGGTCTGCTGAGTCCG-3′, antisense 5′-GTCCATGGGAAGATGTTCTGG-3′; Fgf21 : sense 5′-CTGCTGGGGGTCTACCAAG-3′, antisense 5′-CTGCGCCTACCACTGTTCC-3′; Acox1 : sense 5′-TAACTTCCTCACTCGAAGCCA-3′, antisense 5′-CTGGGCGTAGGTGCCAATTA-3′; Cpt1a : sense 5′-CTCCGCCTGAGCCATGAAG-3′, antisense 5′-CACCAGTGATGATGCCATTCT-3′; Hmgcs2 : sense 5′-ATATGTGGACCAAACTGACCTGG-3′, antisense 5′-ACTGTTTTGACAGCCTTGGAC-3′; Ppar α: sense 5′-AGAGCCCCATCTGTCCTCTC-3′, antisense 5′-ACTGGTAGTCTGCAAAACCAAA-3′; Ppar γ: sense 5′-CTCCAAGAATACCAAAGTGCGA-3′, antisense 5′-GCCTGATGCTTTATCCCCACA-3′; ERdj4 : sense 5′-ATAAAAGCCCTGATGCTGAAGC-3′, antisense 5′-GCCATTGGTAAAAGCACTGTGT-3′; Srebp1c : sense 5′-TGACCCGGCTATTCCGTGA-3′, antisense 5′-CTGGGCTGAGCAATACAGTTC-3′; Fasn : sense 5′-GGCTCTATGGATTACCCAAGC-3′, antisense 5′-CCAGTGTTCGTTCCTCGGA-3′; Acc1 : sense 5′-GATGAACCATCTCCGTTGGC-3′, antisense 5′-CCCAATTATGAATCGGGAGTGC-3′; Scd1 : sense 5′-AGATCTCCAGTTCTTACACGACCAC-3′, antisense 5′-GACGGATGTCTTCTTCCAGGTG-3′; Dgat2 : sense 5′-GCGCTACTTCCGAGACTACTT-3′, antisense 5′-GGGCCTTATGCCAGGAAACT-3′; Sec61 α: sense 5′-TGTCATCTTGCCGGAAATTCA-3′, antisense 5′-CGCATCCAGTAGAACGGGTC-3′. The specificity of each primer pair was confirmed by BLAST analysis as well as its dissociation curve. The CT (cycle threshold) values within the range of 16–30 were considered to be valid for further quantitative use. In addition, the specificity of the primers for detecting Xbp1s mRNA was verified by regular RT–PCR analysis of the total RNA isolated from hepatocytes infected by the adenovirus expressing the unspliced form XBP1u (Ad-XBP1u) or spliced form XBP1s (Ad-XBP1s). The primers could generate a single band for cells infected by Ad-XBP1s but no products for cells infected by Ad-XBP1u (data not shown). Antibodies and immunoblotting p-IRE1α antibody was purchased from Novus Biologicals (NB 100-2323). Antibodies against IRE1α (3294), p-eIF2α (9721), eIF2α (9722), p-Akt (9271), Akt (9272), ACC1 (3662) and Lamin A/C (2032) were all from Cell Signaling. HSP90 (610418) and FAS (610962) antibodies were from BD Biosciences, ATF6α (IMG–273) antibody was from IMGENEX, XBP1s (647501) antibody from Biolegend, PPARα (SC–9000) antibody from Santa Cruz Biotechnology, and α-tubulin (T6199) antibody from Sigma. HSP90 antibody was diluted 1:5,000 for use, α-tubulin antibody was 1:10,000 and PPARα antibody 1:200. All other antibodies were diluted 1:1,000. For immunoblotting, total tissue or cellular lysates were prepared by RIPA buffer (150 mM NaCl, 1% NP-40, 0.5% sodium deoxycholate, 0.1% SDS, 50 mM Tris-HCl, pH 7.4), and nuclear extracts were prepared using NE-PER Nuclear and cytoplasmic extraction kit (Thermo Scientific). Protein extracts were separated by SDS–polyacrylamide gel electrophoresis (SDS–PAGE) and transferred onto a polyvinylidene difluoride (PVDF) membrane filter (Millipore). After incubation with desired antibodies, the blots were developed with Thermo Scientific’s SuperSignal West Pico Chemiluminescent substrate or Millipore’s Immunobilon Western Chemiluminescent HRP substrate. For mobility shift analyses of p-IRE1α, immunoblotting was conducted using the phos-tag gel as described [21] , [22] . Briefly, 50 mM Phos-tag (NARD Institute) and 50 mM MnCl2 (Sigma) were added at 1:100 to the 6% SDS–PAGE gel, which were soaked in 1 mM EDTA for 10 min before transfer onto the PVDF membrane filter. Uncropped scans of the most important immunoblots are shown in Supplementary Fig. 5 . Chromatin immunoprecipitation (ChIP) ChIP assays were performed with the Agarose ChIP kit (Pierce, 26156) following the manufacturer’s instructions. Briefly, hepatocytes, tissues or 293T cells were subjected to cross-linking with 1% formaldehyde. Glycine solution was then added and nuclear extracts were prepared. Chromatin-XBP1s complexes were immunoprecipitated with anti-Flag (Sigma, F3165; diluted 1: 500) or anti-XBP1s (Biolegend, 647501; diluted 1:100) antibodies by incubation at 4 °C for overnight on a rocking platform, followed by incubation with beads from the Agarose ChIP Kit (Pierce) or Protein G-Sepharose beads (GE Health) at 4 °C for 1 h with gentle rocking. After washing 5 times with the washing buffer, the complexes were eluted with the elution buffer from the beads, and were subjected to PCR analysis. The oligonucleotide primers that correspond to the −433 to −220 region (sense 5′-AGCAGCCAATCAGACACTGCCGTCCAG-3′, and antisense 5′-CACCCCTGTCGTGGGACCGTAGCG-3′) or the −1917 to −1750 region (sense 5′-GAACTCAGGACCTACAACCAAGCACCC-3′, and antisense 5′-TCAAAGACAACATTAGTCCATTTTCCTACCCT-3′) of the mouse Ppar α promoter were used. Statistical analysis All data are presented as the mean±s.e.m. Statistical analysis was conducted using unpaired two-tailed t -test, one-way or two-way analysis of variance followed by Bonferroni’s post test with GraphPad Prism 4.0. P <0.05 was considered to be statistically significant. How to cite this article: Shao, M. et al . Hepatic IRE1α regulates fasting-induced metabolic adaptive programs through the XBP1s–PPARα axis signalling. Nat. Commun. 5:3528 doi: 10.1038/ncomms4528 (2014).